Burning vegetation produces cyanohydrins that liberate cyanide and stimulate seed germination Cyanide is well known for its toxicity towards living organisms. Many plants use cyanide as a defensive agent against herbivores, releasing it through the enzymatic hydrolysis of endogenous cyanogenic compounds. At low concentrations, cyanide has been proposed to have a regulatory role in many plant processes including stimulation of seed germination. However, no ecological role for cyanide in seed germination has been established. In the present study, we show that burning plant material produces the cyanohydrin, glyceronitrile. We also show that, in the presence of water, glyceronitrile is slowly hydrolysed to release cyanide that stimulates seed germination of a diverse range of fire-responsive species from different continents. We propose that glyceronitrile serves as an ecological store for cyanide and is an important cue for stimulating seed germination and landscape regeneration after fires. Fire is a global ecological phenomenon known to influence plant growth and diversity in a range of ecosystems [1] , [2] . Smoke derived from burning plant material is a key agent responsible for promoting seed germination following fire [3] and increases seed germination of an estimated 1,200 phylogenetically diverse plant species [4] . Smoke contains thousands of different compounds and there have been many attempts to identify the active compound(s) [5] , [6] , [7] , [8] , [9] , [10] . In 2004, a potent bioactive compound in cellulose- and plant-derived smoke was identified as 3-methyl-2 H -furo[2,3- c ]pyran-2-one ( 1 ) ( Fig. 1a ) [11] , which was recently named karrikinolide (or KAR 1 ) after the Aboriginal Noongar word for smoke, karrik [12] . Smoke-responsive seeds of a large number of species respond to karrikinolide, demonstrating that it is a major contributor to the germination activity of smoke and an ecologically significant germination cue [13] , [14] , [15] . 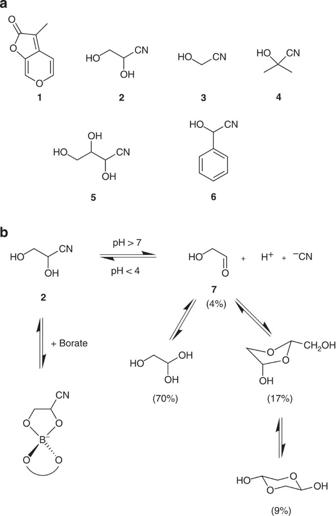Figure 1: Chemical structures and glyceronitrile dissociation. (a) Karrikinolide (1), glyceronitrile (2), glycolonitrile (3), acetone cyanohydrin (4), 2,3,4-trihydroxybutyronitrile (5) and mandelonitrile (6). (b) Equilibrium at different pH of glyceronitrile (2) with glycolaldehyde (7) and hydrogen cyanide as well as the equilibrium possible with borate minerals41and the equilibrium of glycolaldehyde with hydrated and dimeric species that are known to form in aqueous solutions (parentheses values indicate relative amounts at equilibrium in aqueous solutions40). Figure 1: Chemical structures and glyceronitrile dissociation. ( a ) Karrikinolide ( 1 ), glyceronitrile ( 2 ), glycolonitrile ( 3 ), acetone cyanohydrin ( 4 ), 2,3,4-trihydroxybutyronitrile ( 5 ) and mandelonitrile ( 6 ). ( b ) Equilibrium at different pH of glyceronitrile ( 2 ) with glycolaldehyde ( 7 ) and hydrogen cyanide as well as the equilibrium possible with borate minerals [41] and the equilibrium of glycolaldehyde with hydrated and dimeric species that are known to form in aqueous solutions (parentheses values indicate relative amounts at equilibrium in aqueous solutions [40] ). Full size image However, our early research on seeds of smoke-responsive taxa from the global biodiversity hotspot of southwest Australia identified an iconic species with seeds that do not respond to karrikinolide, despite the well-documented response of these seeds to plant-derived smoke [16] . The species, Anigozanthos manglesii (commonly known as the red and green kangaroo paw), is a member of the ancient Gondwanan family Haemodoraceae, which comprises highly divergent and relictual taxa in southwest Australia [17] . Most species of this genus produce smoke-responsive seeds [18] , [19] and the inactivity of karrikinolide with A. manglesii seeds suggested that a separate bioactive compound(s) is present in smoke. We now report a new major germination stimulant in smoke that initiates the germination of A. manglesii and several other smoke-responsive species. The compound has been isolated from plant-derived smoke and confirmed by synthesis as the cyanohydrin, glyceronitrile. Several related cyanohydrins also stimulate germination, and we demonstrate that the activity of these compounds is due to the spontaneous release of cyanide, suggesting a new ecological role for cyanide in the post-fire regeneration of diverse plant communities. Detection and isolation of the active compound Our investigation into the A. manglesii germination stimulant revealed that it was not produced by the burning of cellulose, a substrate that is known to produce karrikinolide [11] . Instead, combustion of plant material was required to obtain smoke-water extracts that stimulated the germination of A. manglesii ( Fig. 2 ). The active compound was also much more polar than karrikinolide ( 1 ), because it was not extractable from smoke water with dichloromethane and was not retained by a C 18 reversed-phase silica sorbent. Conveniently, these results led to a method to simplify the smoke-water mixture by eluting the filtered solution through a column of C 18 reversed-phase silica. The non-polar organic compounds present, including karrikinolide, were retained on the column, whereas the more polar compounds, including the A. manglesii stimulant, were eluted in the aqueous fraction. Exhaustive extraction of this aqueous fraction with ethyl acetate enabled the majority of the germination activity to be concentrated into the organic fraction. 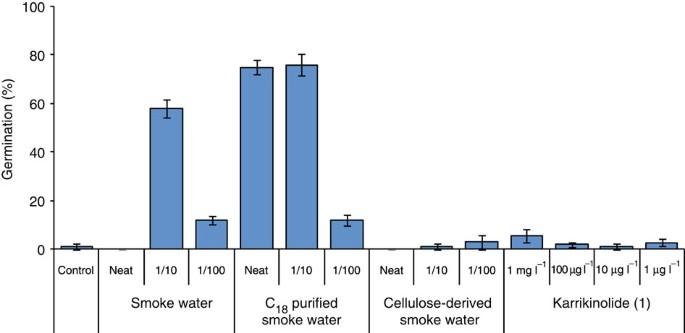Figure 2: Germination ofA. manglesii. Comparison ofA. manglesiigermination response with smoke water, C18purified smoke water, cellulose-derived smoke water and karrikinolide (1). Values are means of three replicates±s.e. Figure 2: Germination of A. manglesii . Comparison of A. manglesii germination response with smoke water, C 18 purified smoke water, cellulose-derived smoke water and karrikinolide ( 1 ). Values are means of three replicates±s.e. Full size image Semi-preparative HPLC of the ethyl acetate fraction using a C 18 reversed-phase sorbent resulted in further purification. The active component eluted between 4–5 min, and was found to have no significant ultraviolet absorption ( Supplementary Fig. S1 ). This active fraction was subjected to normal phase HPLC using a diol column, which resulted in good retention of the analyte according to the bioassay ( Supplementary Fig. S2 ). Preparative separation using this method, followed by further separation using the diol column resulted in the purification of a compound with significant germination activity towards A. manglesii . Using 1 H, 13 C and 2D nuclear magnetic resonance (NMR) spectroscopy, the compound was identified as the cyanohydrin, 2,3-dihydroxypropanenitrile ( 2 ) ( Fig. 1a ; Supplementary Fig. S3 ), which is also known as glyceronitrile. Confirmation of germination activity Testing of an authentic racemic sample of glyceronitrile [20] against seeds of A. manglesii and the South African species Rhodocoma arida (Restionaceae), which also responds poorly to karrikinolide [11] , confirmed that glyceronitrile ( 2 ) was bioactive with both species ( Fig. 3a,b ). To determine the relative activity of the enantiomers of glyceronitrile, their synthesis from ( S) - and ( R) -glyceraldehyde [21] , [22] , respectively, was undertaken [23] . Both enantiomers were equally active in germination activity with A. manglesii ( Supplementary Fig. S4 ) and subsequent enantioselective HPLC of the smoke-derived compound confirmed that a racemic mixture was isolated. 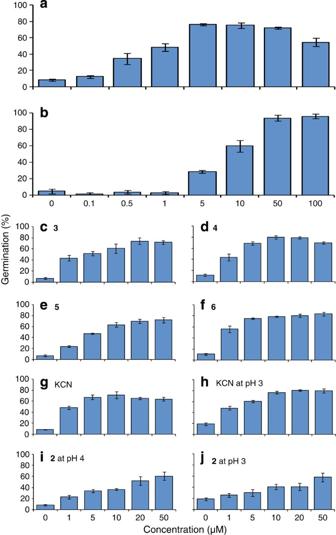Figure 3: Testing of cyanohydrins and cyanide for germination promotion. Comparison of the germination response of different concentrations of glyceronitrile (2) with (a)A. manglesiiand (b)R. arida. Germination ofA. manglesiiincubated with different concentrations of (c) glycolonitrile (3), (d) acetone cyanohydrin (4), (e) 2,3,4-trihydroxybutyronitrile (5), (f) mandelonitrile (6), (g) KCN, (h) KCN at pH 3 (1 mM HCl/glycine buffer), (i) glyceronitrile (2) at pH 4 (1 mM acetic acid/sodium acetate), and (j) glyceronitrile (2) at pH 3 (1 mM HCl/glycine). Water (0 μM) served as the control in each experiment and values are means of three replicates±s.e. KCN, potassium cyanide. Figure 3: Testing of cyanohydrins and cyanide for germination promotion. Comparison of the germination response of different concentrations of glyceronitrile ( 2 ) with ( a ) A. manglesii and ( b ) R. arida . Germination of A. manglesii incubated with different concentrations of ( c ) glycolonitrile ( 3 ), ( d ) acetone cyanohydrin ( 4 ), ( e ) 2,3,4-trihydroxybutyronitrile ( 5 ), ( f ) mandelonitrile ( 6 ), ( g ) KCN, ( h ) KCN at pH 3 (1 mM HCl/glycine buffer), ( i ) glyceronitrile ( 2 ) at pH 4 (1 mM acetic acid/sodium acetate), and ( j ) glyceronitrile ( 2 ) at pH 3 (1 mM HCl/glycine). Water (0 μM) served as the control in each experiment and values are means of three replicates±s.e. KCN, potassium cyanide. Full size image Further evaluation of glyceronitrile was undertaken with seeds of a range of species known to be responsive to smoke, with a focus on species of Australian Haemodoraceae and other key smoke-responsive species from Australia, South Africa and North America. In addition, the stimulatory effects of smoke water and karrikinolide were tested for comparison. Germination of seeds of a second accession of A. manglesii , as well as the closely related species Anigozanthos humilis and Anigozanthos viridis , was significantly greater ( P <0.05) in the presence of glyceronitrile ( Fig. 4 ; Supplementary Table S1 ) when compared with seeds incubated in water or karrikinolide solution. Seeds of three other Western Australian species ( Andersonia latiflora , Conostylis candicans and Ficinia nodosa ) that had significantly greater ( P <0.05) germination when incubated in smoke water also had significantly greater germination when incubated with either glyceronitrile or karrikinolide ( Fig. 4 ). Furthermore, smoke-responsive seeds of the North American species Emmenanthe penduliflora and a second accession of the South African R. arida also had significantly greater ( P <0.05) germination when incubated with glyceronitrile. 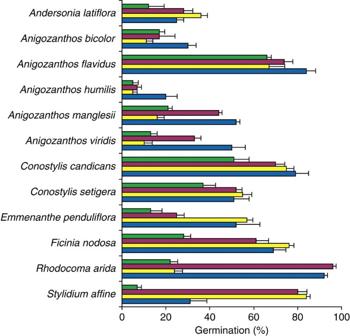Figure 4: Germination response of glyceronitrile. Selected Australian Haemodoraceae and key smoke-responsive species from Australia, South Africa and North America. Species were incubated with water only (green), 1/10 diluted smoke water (maroon), 1 μM karrikinolide (1, yellow) and 50 μM glyceronitrile (2, blue). Values are means of three replicates±s.e. Numerical values and statistical analysis are presented inSupplementary Table S1. Figure 4: Germination response of glyceronitrile. Selected Australian Haemodoraceae and key smoke-responsive species from Australia, South Africa and North America. Species were incubated with water only (green), 1/10 diluted smoke water (maroon), 1 μM karrikinolide ( 1 , yellow) and 50 μM glyceronitrile ( 2 , blue). Values are means of three replicates±s.e. Numerical values and statistical analysis are presented in Supplementary Table S1 . Full size image Glyceronitrile mode of action Cyanohydrins are widespread in nature and are formed by hydrolysis of cyanogenic glycosides, which are present in over 3,000 plant species [24] . Spontaneous decomposition of the cyanohydrin or enzymatic catalysis by an α-hydroxynitrile lyase can yield hydrogen cyanide and an aldehyde or a ketone [25] . Hydrogen cyanide or solutions of cyanide can stimulate the germination of seeds of different plant species [26] , [27] , [28] , [29] , [30] and different aldehydes and ketones can also promote seed germination [31] . The dormancy-breaking effect of cyanides can be elicited by continuous contact at low doses or by short exposure times (ca. 3 h) at relatively high concentration (ca. 1 mM) followed by removal of the cyanide source [32] , [33] . We tested KCN at various concentrations in a continuous incubation mode and found that it promoted the germination of A. manglesii at concentrations similar to those found effective for glyceronitrile ( Fig. 3g ). Furthermore, the cyanohydrin analogues glycolonitrile ( 3 ), acetone cyanohydrin ( 4 ), 2,3,4-trihydroxybutyronitrile ( 5 ) and mandelonitrile ( 6 ) ( Fig. 1a ) were also active ( Fig. 3c-f ). In contrast, glycolaldehyde ( 7 ) showed no germination promoting ability ( Supplementary Fig. S5 ). Taken together, these results suggest that the cyanohydrins are acting by releasing cyanide and that cyanide, rather than the aldehyde, is the active germination stimulant. However, at this point, it was not clear whether the spontaneous or the enzymatic generation of cyanide was operating. Aqueous solutions of glyceronitrile ( 2 ) are known to be in equilibrium with glycolaldehyde ( 7 ) and hydrogen cyanide at pH 7 and above, whereas below pH 4, glyceronitrile is relatively stable ( Fig. 1b ) [34] . Fresh, unbuffered aqueous solutions of glyceronitrile were found to contain very low levels of cyanide ( Fig. 5a ) [35] . However, over a period of 12 days, the time needed for A. manglesii seeds to complete germination, the amount of free cyanide increased and approached that of the cyanide standards ( Fig. 5a ). When glyceronitrile was buffered at low pH the amount of free cyanide detected was significantly lower ( Fig. 5b ). For solutions of glyceronitrile incubated in the presence of whole seeds or a seed extract of A. manglesii , the concentration of cyanide remained similar to that in solutions containing only glyceronitrile, and decreased after 4 days, presumably as the cyanide was consumed by the seeds ( Fig. 5c ). When compared with racemic mandelonitrile in the presence of α-hydroxynitrile lyase, naturally present in almonds ( Prunas amygdalus , Rosaceae), in the presence of racemic mandelonitrile ( 6 ), where the natural substrate is ( R )-mandelonitrile [24] , significant conversion to free cyanide and benzaldehyde was noted within minutes ( Fig. 5d ). A similar time-scale experiment with an A. manglesii seed extract revealed no increase in cyanide levels following the addition of glyceronitrile ( Fig. 5d ). In addition, germination activity of glyceronitrile at low pH showed that the solutions had reduced germination activity towards A. manglesii ( Fig. 3i,j ), yet pH 3 buffered cyanide solutions retained high activity ( Fig. 3h ). Furthermore, testing of the enantiomers of glyceronitrile for germination activity under different pH conditions failed to indicate any enantioselective activity, which would be expected for an enzyme-catalysed reaction ( Supplementary Fig. S4 ). Thus, these results indicate that enzymatic degradation is not significant and that the spontaneous production of cyanide is responsible for the activity observed for glyceronitrile and related cyanohydrins. 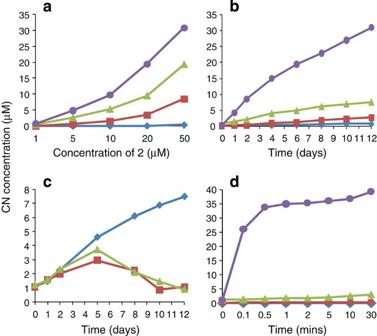Figure 5: Colorimetric detection of cyanide in glyceronitrile (2) solutions. (a) Concentration of free cyanide detected in solutions of glyceronitrile (2) in water only at different concentrations and over a period of 0 (blue diamonds), 2 (red squares), 6 (green triangles) and 12 (purple circles) days. (b) Concentration of cyanide detected in a 50 μM solution of glyceronitrile (2) at pH 3 (blue diamonds), pH 4 (red squares), pH 4.6 (green triangles) and water only (purple circles) over a period of 12 days. (c) Concentration of cyanide detected in a 50 μM solution of glyceronitrile (2) at pH 4.6 (blue diamonds), in the presence ofA. manglesiiwhole seeds (red squares) or anA. manglesiiaqueous seed extract (green triangles) over a period of 12 days. (d) Concentration of cyanide detected in a 50 μM solution of glyceronitrile (2) at pH 4.6 (blue diamonds) and in the presence of anA. manglesiiseed extract (red squares) over 30 min compared with the cyanide detected in a 50 μM solution of mandelonitrile (6) at pH 4.6 (green triangles) and in the presence of an aqueous extract of almonds containing mandelonitrile lyase (purple circles). Figure 5: Colorimetric detection of cyanide in glyceronitrile (2) solutions. ( a ) Concentration of free cyanide detected in solutions of glyceronitrile ( 2 ) in water only at different concentrations and over a period of 0 (blue diamonds), 2 (red squares), 6 (green triangles) and 12 (purple circles) days. ( b ) Concentration of cyanide detected in a 50 μM solution of glyceronitrile ( 2 ) at pH 3 (blue diamonds), pH 4 (red squares), pH 4.6 (green triangles) and water only (purple circles) over a period of 12 days. ( c ) Concentration of cyanide detected in a 50 μM solution of glyceronitrile ( 2 ) at pH 4.6 (blue diamonds), in the presence of A. manglesii whole seeds (red squares) or an A. manglesii aqueous seed extract (green triangles) over a period of 12 days. ( d ) Concentration of cyanide detected in a 50 μM solution of glyceronitrile ( 2 ) at pH 4.6 (blue diamonds) and in the presence of an A. manglesii seed extract (red squares) over 30 min compared with the cyanide detected in a 50 μM solution of mandelonitrile ( 6 ) at pH 4.6 (green triangles) and in the presence of an aqueous extract of almonds containing mandelonitrile lyase (purple circles). Full size image Natural presence of glyceronitrile in smoke water To confirm that glyceronitrile was present in smoke water and not formed during purification, the cyanide content was tested. No free cyanide was detected in smoke water (pH 2.8) that had been prepared in 2006. The amount of glyceronitrile present was quantified by derivatization with N,O -bis(trimethylsilyl)trifluoroacetamide (BSTFA) and analysis using gas chromatograph–mass spectrometry (GC–MS). The results showed that 300 (±30) μM of glyceronitrile was present in the smoke water used in this study. Furthermore, 46 (±3) μM of glycolonitrile ( 3 ) was also detected by comparison with an authentic sample. In a smoke-water sample that had been generated by burning a mixture of fresh and dried shoot material collected from local bushland [18] , [36] , 190 (±17) μM of glyceronitrile and 8.9 (±0.9) μM of glycolonitrile, were also detected. Although the source of plant material, combustion duration and temperature are likely to influence the amounts present, these results indicate that in a 10% (v/v) diluted sample, typically used for seed germination studies, the concentration of glyceronitrile is within the range (5–50 μM) expected to promote seed germination. As the reaction of cyanide with aldehydes or ketones to form cyanohydrins does not occur below pH 5 (ref. 34 ), these results suggest that glyceronitrile (and glycolonitrile) is formed during combustion. As glyceronitrile exists in equilibrium with cyanide and glycolaldehyde, it is reasonable to envisage that when diluted (for example, by rain) or in the presence of seeds at physiological pH, free cyanide will be slowly released in sufficient quantity to stimulate seed germination. Cyanide is generally regarded as an important signaling molecule for a variety of plant processes, including seed germination [25] , and some seeds are known to evolve hydrogen cyanide during the germination process [37] , [38] . The mode of action of cyanide in stimulating seed germination remains unclear but is thought to involve reactive oxygen species [32] , [39] . It has also been proposed that cyanide acts at an initial step in dormancy alleviation and nitrogen oxide is required at a later step [33] . This is interesting given that nitrogen oxides (NO and NO 2 ) have previously been proposed as germination-active components of smoke and can stimulate the germination of E. penduliflora [8] . However, the ecological relevance and persistence of nitrogen oxides in natural settings has been questioned [9] . Our results show that glyceronitrile is stable for a number of years and can release quantitative amounts of cyanide under appropriate conditions. This sustained release of cyanide is most likely driven by the hydration and dimerization of its co-product, glycolaldehyde ( 7 ), processes that are known to predominate in aqueous solutions [40] ( Fig. 1b ). In addition to acting as a store of hydrogen cyanide, glyceronitrile also contains a glycol (1,2-dihydroxyl) functionality that is known to be stabilized by minerals containing borate [41] ( Fig. 1b ), which could explain the possible ecological persistence of this compound deposited on soil following a fire event. Furthermore, the glycol functionality is known to form intramolecular hydrogen bonding arrangements [42] , which may restrict spontaneous cyanide release compared with other cyanohydrins ( Fig. 5d ) [35] . In summary, our discovery of glyceronitrile ( 2 ) as a new major germination stimulant in smoke, acting through the slow release of cyanide, provides for the first time a potential ecological context to the seed germination enhancing properties of cyanide. It also offers new opportunities for releasing seed dormancy in many species, especially those that are known to respond to cyanide. In addition, intriguing possibilities exist to understand why some taxa, exemplified by Australian Anigozanthos spp. and African R. arida , respond only to glyceronitrile, some exemplified by Conostylis spp. and E. penduliflora , respond to both karrikinolide and glyceronitrile, and yet others, such as Stylidium affine , respond better to karrikinolide. The different chemical properties of karrikinolide ( 1 ) and glyceronitrile ( 2 ) suggest that plant seeds may have evolved independent, or even multiple, mechanisms to detect and respond to wildfires, and unravelling these responses may provide a basis for understanding evolutionary adaptations of plants to fire. General experimental 1 H and 13 C NMR spectra were obtained on a Bruker AV600 (600 MHz for δ H and 150.9 MHz for δ C ) spectrometer using hexadeuteroacetone ((CD 3 ) 2 CO) as solvent and residual (CH 3 ) 2 CO ( δ H 2.04) or (CD 3 ) 2 CO ( δ C 29.8) as internal standards. GC–MS was conducted using an Agilent 5973 mass selective detector. HPLC was conducted using a Hewlett Packard 1050 HPLC system equipped with a multiple wavelength detector. Semi-preparative HPLC was conducted using a Rainin Dynamax SD-300 solvent delivery system. Optical rotation was conducted using a Perkin-Elmer 141 polarimeter. Ultraviolet-Vis experiments were conducted with a Perkin-Elmer Lambda 25 spectrophotometer. Isopropanol, acetonitrile and hexane were of HPLC grade and used without further purification. Acetonitrile was dried by storage over 3 Å molecular sieves. Other solvents used were distilled before use. Milli-Q water was obtained by filtration of deionised water through a Milli-Q ultrapure water system (Millipore). N,O -BSTFA containing 1% trimethylchlorosilane, glycolonitrile ( 3 ) and glycolaldehyde dimer were purchased from Sigma-Aldrich. Plant-derived smoke water [36] and cellulose-derived smoke water [10] were prepared as previously reported and frozen at −18 °C until use. A. manglesii bioassay A. manglesii D. Don. (Haemodoraceae) seed was from wild-sourced plants naturally seeding in bushland at Kings Park and Botanic Garden, Perth in 1999. After a period of dry after-ripening (ca. 1 yr), seeds were sealed in laminated aluminium foil bags and stored at −18 °C prior to germination experiments. For testing, three replicates of 20–30 seeds were vacuum sterilized [36] and added to ultraviolet-sterilised petri dishes (90 mm), containing two Whatman No.1 filter papers (7 cm) moistened with the test solution (2.7 ml). Milli-Q-purified water was used as a control for each experiment, and dilutions of each sample were used to ensure the optimum concentration range for activity. Petri dishes were sealed with parafilm and incubated in the dark at 20±1 °C. The seeds were scored for germination after 12 days of incubation. Testing of other species Seeds of Anigozanthos bicolor Endl. (Haemodoraceae), A. flavidus DC. (Haemodoraceae), A. humilis Lindl. (Haemodoraceae), A. manglesii D.Don. (Haemodoraceae), A. viridis Endl. (Haemodoraceae), C. aculeata R.Br. (Haemodoraceae), C. candicans Endl. (Haemodoraceae), Conostylis setigera R.Br. (Haemodoraceae), Andersonia latiflora (F.Muell.) Benth. (Ericaceae), Ficinia nodosa (Rottb.) Goetgh., Muasya & D.A.Simpson (Cyperaceae) and Stylidium affine Sond. (Stylidiaceae) were sourced from wild populations in southwest Western Australia. Seeds were of varied age but did not exceed 3 years of age. Seeds of Emmenanthe penduliflora Benth. (Hydrophyllaceae) were received from California State University, USA. Seeds of Rhodocoma arida H.P. Linder and J.H. Vlok (Restionaceae) were sourced from wild populations and supplied by Cape Seeds, Cape Town, South Africa. All seeds were dried at 15 °C and 15% relative humidity upon receipt, hermetically sealed in laminated aluminium foil bags and stored at −18°C prior to germination experiments. Four replicates of 25 seeds were sterilized in 2% calcium hypochlorite (Ca(OCl) 2 ), rinsed in sterile de-ionised water and sown in 90 mm Petri dishes containing two Whatman No. 1 filter papers (7 mm) and irrigated with sterile de-ionized water (control), glyceronitrile (50 μM), karrikinolide (1 μM) or smoke water 1:10 (v/v). Petri dishes were placed at 15 °C in incubators with a daily 12-h photoperiod of 30 μmol m −2 s −1 400–700 nm, cool-white fluorescent light. Seeds were scored weekly for germination for 4 weeks. A seed was considered germinated upon radicle emergence >2 mm. Statistical analysis Germination data were analysed for statistical significance by analysis of variance using Genstat 9th Ed (Lawes Agricultural Trust). Percentage values for germination were arcsine-transformed prior to analysis (untransformed data appears in all figures). Fisher's least significant difference at the 5% level ( P <0.05) was used to separate means and determine significant differences between treatments. C 18 purification and extraction of smoke water Smoke water (20 l) was prepared from combustion of agricultural feed straw (oaten hay) [43] using the apparatus previously described [18] . Smoke water (2 l) was filtered (32 cm, Whatman No. 1) and added to a vacuum-assisted chromatography column (60×4.5 cm id) packed with C 18 reversed-phase silica (100 g, 60 μm, Grace-Davison SPE HC C18 (633N)). The smoke water was separated into 2 fractions: the C 18 non-retained (aqueous fraction) and the C 18 retained fraction, which was eluted with methanol (300 ml). This was repeated five times and the combined C 18 non-retained fraction was exhaustively extracted with ethyl acetate, combined and evaporated to dryness under reduced pressure to give a yellow oil (2.5 g from 10 l smoke water). C 18 semi-preparative HPLC The ethyl acetate extract (2.5 g) was dissolved in 5% acetonitrile/water (100 ml) and a sample (10 ml) was separated by semi-preparative HPLC using a 250×22 mm i.d., 5 μm, Apollo C 18 reversed-phase column (Grace-Davison). The column was eluted at 20 ml per min with 5% acetonitrile/water for 20 min, increasing to 60% acetonitrile/water for 15 min. Fractions were collected every min for 30 min and repeated ten times with similar fractions combined. A small sample (ca. 300 μl) was taken and purged to dryness before adding milli-Q water (10 ml) for testing neat and at 1/10 dilution with the A. manglesii bioassay. Normal phase (diol) HPLC The active fraction from C 18 semi-preparative HPLC (fraction 5, corresponding to 4–5 min retention time) was separated by normal phase HPLC using a 250×4 mm i.d., 5 μm, Lichrospher 100 Diol column (Merck). The column was eluted at 1 ml per min with 5% isopropanol/hexane increasing to 50% isopropanol/hexane over 25 min and held for 5 min. Fractions were collected every min and a small sample (ca. 150 μl) was taken and purged to dryness under nitrogen before adding milli-Q water (10 ml) for testing neat with the A. manglesii bioassay. The active fraction (fraction 14) was separated further using the same diol column and eluted with a mobile phase of 15% isopropanol/hexane. Fractions were collected every min and a small sample (ca. 150 μl) was taken and purged to dryness before adding milli-Q water (10 ml) for testing neat with the A. manglesii bioassay. The active fraction (fraction 12) was evaporated to dryness (9.4 mg) and analysed by 1 H, 13 C and two-dimensional NMR spectroscopy ( 1 H- 1 H COSY, HSQC, HMBC). The compound was identified as 2,3-dihydroxypropanenitrile ( 2 ) by comparison with literature parameters [20] . For 2 : 1 H NMR (600 MHz, D 6 -acetone) δ H 4.58 (t, J =5.6 Hz, 1H), 3.74 (d, J =5.6 Hz, 2H). 13 C NMR (150.9 MHz, D 6 -acetone) δ C 120.4 (CN), 64.6 (CH 2 ), 63.3 (CH). Synthesis Karrikinolide ( 1 ) [44] , glyceronitrile ( 2 ) [20] , 2,3,4-trihydroxybutyronitrile ( 4 ) [34] , acetone cyanohydrin ( 5 ) [45] and mandelonitrile ( 6 ) [46] were prepared according to literature procedures. Synthesis of the ( R )- and ( S )-enantiomers of 2 were achieved from ( S )- and ( R )-glyceraldehyde [21] , [22] respectively following the method of Chelucci et al . [23] ( S )-2,3-dihydroxypropanitrile: [α] D =+15.5° ( c 1.0, MeOH), +31.2° ( c 1.0, H 2 O), ( R )-2,3-dihydroxypropanitrile: [α] D =−15.4° ( c 0.8, MeOH). Enantioselective HPLC A sample of the synthetic enantiomers (ca. 1 mg) of 2 were converted into their acetate derivatives using acetic anhydride (200 μl) and pyridine (200 μl) by heating at 50 °C for 10 min. The solutions were purged to dryness under a stream of N 2 and reconstituted in dry acetonitrile (1 ml). The acetylated compounds were analysed for enantiomeric excess (ee) by enantioselective HPLC using a 250×4.6 mm i.d., 5 μm Chiracel OD-H column (Daicel) and an injection volume of 20 μl. The column was eluted at 0.8 ml per min with 20% isopropanol/hexane, and peaks were detected at an ultraviolet wavelength of 210 nm. R t ( R -diacetate)=16.7 min, R t ( S -diacetate)=17.8 min. GC–MS analysis of smoke water and glyceronitrile Smoke water (straw- or plant-derived) was purified through a Waters Sep-pak ® (Classic C18 cartridge, WAT051910). The smoke water (10 ml) was eluted through the Sep-pak followed by Milli-Q water (5 ml) and the eluates were combined and evaporated to dryness to give an oily residue (straw=54.2 mg, plant=33.4 mg). A sample of the extracts (1/10) and 2 (1.0 mg) were derivatized using N,O -BSTFA containing 1% trimethylchlorosilane (200 μl) and pyridine (200 μl) and heated at 60 °C for 20 min. The resulting solutions were diluted with dry acetonitrile before analysis by GC–MS (for SW diluted to 1 ml, for 2 diluted to 0.1, 0.05, 0.01 and 0.005 mg/ml for quantification). Separation was achieved using a 30 m×0.25 mm i.d., 0.25 μm, BPX-5 column (SGE) with UHP helium as the carrier gas (1 ml per min). The initial oven temperature was set to 40 °C and held for 1 min before increasing at 7 °C per min to 280 °C and held for 10 min (inlet temperature 280 °C; transfer line 280 °C). The ion source was set at 200 °C and the spectrometer was set to record between 45 and 400 amu. For quantification, the samples and standards were analysed in selective ion monitoring mode using m/z 117 (and qualifier ion m/z 201) for 2 . Similarly, a sample of glycolonitrile ( 3 ) was derivatized and analysed as above using SIM of m/z 114 (and qualifier ion m/z 84) for quantification. GC–MS (EI), mass (relative abundance): For 2 , (2×TMS, R t =12.32 min) m/z 216 (10, M-15), 201 (35), 186 (13), 117 (100), 103, (22), 100 (14), 73 (67). For 3 , (TMS, R t =7.01 min) m/z 114 (100, M-15), 84 (94). Colorimetric cyanide detection Solutions (100 ml) of 2 were prepared at different concentrations (1–50 μM) in either H 2 O, 1 or 10 mM (for enzyme related assays, Fig. 5c,d ) acetic acid/sodium acetate buffer (pH 4 or 4.6) or 1 mM HCl/glycine buffer [47] (pH 3). Samples were analysed for CN content using essentially the method of Selmar et al . [35] with some modifications. Briefly, to a sample (10 ml) from each solution was added the chlorosuccinimide reagent (5 ml of 0.25 g N -chlorosuccinimide/2.5 g succinimide in 1 l H 2 O) and left to stand for 2 min. The barbituric acid/pyridine reagent (1 ml of 15 g barbituric acid/150 ml pyridine/350 ml H 2 O) was added and left to stand for 10 min before ultra violet absorbance measurements at 580 nm. Using this method cyanide could be detected at concentrations as low as 0.2 μM. How to cite this article : Flematti, G. R. et al . Burning vegetation produces cyanohydrins that liberate cyanide and stimulate seed germination. Nat. Commun. 2:360 doi: 10.1038/ncomms1356 (2011).